Visualization and quantification of transition metal atomic mixing in Mo1−xWxS2single layers The alloying behaviour of materials is a well-known problem in all kinds of compounds. Revealing the heteroatomic distributions in two-dimensional crystals is particularly critical for their practical use as nano-devices. Here we obtain statistics of the homo- and heteroatomic coordinates in single-layered Mo 1− x W x S 2 from the atomically resolved scanning transmission electron microscope images and successfully quantify the degree of alloying for the transition metal elements (Mo or W). The results reveal the random alloying of this mixed dichalcogenide system throughout the chemical compositions ( x =0 to 1). Such a direct route to gain an insight into the alloying degree on individual atom basis will find broad applications in characterizing low-dimensional heterocompounds and become an important complement to the existing theoretical methods. Layered semiconductors TX 2 (T=Mo, W; X=S, Se, Te) are interesting both from a fundamental scientific and a technological point of view, because of their peculiar structural properties. In particular, the as-crystallized two-dimensional (2D) layered structure can impart substantial anisotropy, and scientists have made an effort to acquire a better insight into the fundamental physics of these compounds [1] , [2] , [3] . The materials have also been investigated extensively because of their possible practical applications such as efficient electrodes in photoelectrochemical solar cells [4] , [5] , [6] , catalysts in industrial applications and secondary batteries [7] , [8] , [9] , and solid-state lubricants [10] , [11] , [12] . Several studies concerning the preparation and characterization of Mo 1− x W x S 2 compounds have been reported [13] , [14] , [15] , [16] , [17] . The X-ray diffraction studies confirmed that Mo 1− x W x S 2 compounds synthesized directly from the constituent elements crystallize in a layered structure with hexagonal symmetry [13] , [14] . The thermal decomposition of a thiometallate solid solution (NH 4 ) 2 Mo 1− x W x S 4 in an inert or hydrogen atmosphere yields the formation of Mo 1− x W x S 2 nanotubes and related structures [15] , [16] , [17] . Using piezoreflectance measurements in the vicinity of the direct band edge, it was determined that the transition energies vary smoothly with the tungsten composition x in Mo 1− x W x S 2 compounds [18] . Recently, the indirect to direct alteration of the optical bandgap [19] , [20] and phonon frequency shift [21] , when the MoS 2 thickness decreases to single-layer thickness, have been observed. The single-layer MoS 2 has thus become an appealing material in the area of optoelectronic devices [22] , and the unique properties of MoS 2 can be extended further to various compositions of Mo 1− x W x S 2 to obtain more diverse electronic properties. An understanding of the atomic distributions in mixed Mo 1− x W x S 2 compounds should be a prerequisite for the control of their physical and chemical properties for bandgap engineering or their edge-structure-related catalytic behaviours [23] , [24] . In this work, we performed the direct visualization of the atomic species Mo and W in Mo 1− x W x S 2 compounds, clearly showing how the two elements can be mixed in a single layer. Scanning transmission electron microscope (STEM) annular dark-field (ADF) has already proved its efficiency for imaging 2D crystals such as graphene [25] , h -boron nitride [26] , [27] , WS 2 (ref. 28 ) and MoS 2 (ref. 29 ) with edges, defects or substitutions. Here the STEM-ADF method can be extended to count the neighbouring atoms of two transition metal components that show either mutual attraction or repulsion of the constituent species. The alloying behaviour thus obtained at individual atom basis can be a good contrast to theoretical study such as Monte–Carlo method which statistically treats the alloying properties of the entire system [30] . Observation of mixed Mo 1− x W x S 2 layers A series of mixed Mo 1− x W x S 2 compounds was prepared by the chemical-vapour transport method [18] from the starting materials for compositions with x =0, 0.2, 0.5, 0.8, and 1. The as-grown crystals were cleaved using scotch tape and transferred onto a microscopy grid made of gold Quantifoil [31] . Although a few layer regions are dominant in the cleaved specimens, single-layered regions can be easily found with a discrete atomic contrast (see Supplementary Fig. S1 ). 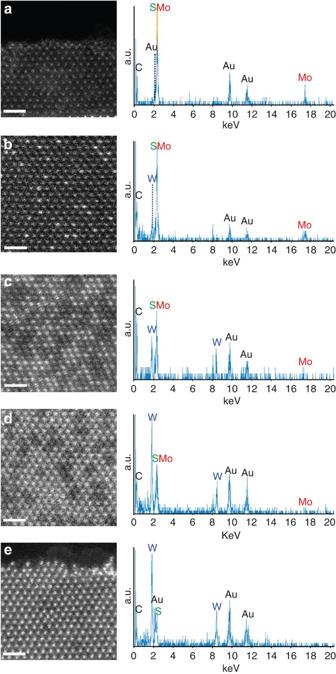Figure 1: STEM-ADF images together with EDX analyses. (a–e) A series of ADF images of Mo1−xWxS2single layers (x=0, 0.2, 0.5, 0.8 and 1 for starting materials), showing the disordered atomic configurations for the two elements throughout the mixture compositions. The brighter spots correspond to the W atom sites and the less bright ones to the Mo sites. Sulphur atoms are not resolved here. The corresponding EDX spectra are also shown on the right, confirming the monotonically increasing W content (a–e). The Au peaks originate to the used STEM specimen grid (Quantifoil, ref.31). Scale bar, 1 nm. Figure 1 shows a series of STEM-ADF images together with the energy dispersive X-ray spectrometry (EDX) analyses of the obtained materials ( x =0, 0.2, 0.5, 0.8 and 1). It is seen that brighter and less bright spots are clearly resolved in the ADF images and that the fraction of brighter spots increases monotonically with increasing x . The different intensities in the ADF images correspond to the two distinct transition metal atoms, namely Mo and W, while the sulphur atoms are not always visible because of the possible inclinations of the layers with respect to the direction of the incident electron beam [28] . Figure 1: STEM-ADF images together with EDX analyses. ( a – e ) A series of ADF images of Mo 1− x W x S 2 single layers ( x =0, 0.2, 0.5, 0.8 and 1 for starting materials), showing the disordered atomic configurations for the two elements throughout the mixture compositions. The brighter spots correspond to the W atom sites and the less bright ones to the Mo sites. Sulphur atoms are not resolved here. The corresponding EDX spectra are also shown on the right, confirming the monotonically increasing W content ( a – e ). The Au peaks originate to the used STEM specimen grid (Quantifoil, ref. 31 ). Scale bar, 1 nm. Full size image Discrimination of Mo and W atoms To discriminate the W and Mo metal atoms in the mixed Mo 1− x W x S 2 layers, we performed atomically resolved electron energy loss spectroscopy (EELS) analysis as well as quantitative simulation of the ADF profiles. 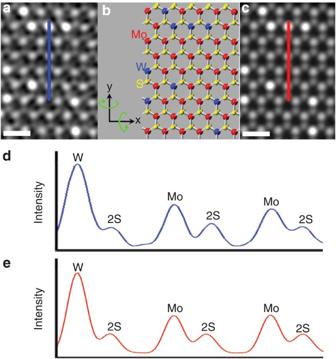Figure 2: Discrimination of Mo and W atoms. (a) An ADF image of a Mo1−xWxS2single layer withx=0.2 (filtered), in which the atomic positions of sulphur are also visible. (b,c) Modelled structure and simulated ADF image (red: Mo, blue: W, yellow: S). Note that the two sulphur atoms are overlapped with a small inclination of (5° in x axis and 6° in y axis). (d,e) Profiles of the experimental and simulated ADF counts for lines indicated inaandc. They confirm the W, Mo and 2S atomic sites, that is, the brighter spots correspond to W and the less bright ones to Mo. Note that a fast Fourier transform smoothing applied might result in an image contrast variation at most 4%. An absorption potential approach using a multislice calculation with the Mactempas software is used in the simulation profile. Scale bar, 0.5 nm. Figure 2 shows the quantitative analysis for the ADF image of a mixed Mo 1− x W x S 2 layer ( x =0.2). The experimental ADF profile along with the blue line in Fig. 2a shows a perfect match with the simulated one (red line in Fig. 2c ) in Fig. 2d , respectively. The possible inclination of the layer (5° in the x axis and 6° in the y axis, shown in Fig. 2b ), which may cause a non-negligible variation in the ADF intensity (especially on the sulphur atomic sites) was taken into account. This atomically resolved ADF image clearly proves that the W and Mo atoms share the metal atom sites, while the sulphur atoms are always paired in the trigonal lattice (modelled in Fig. 2b ). Although the 2H stacking of 3 (or 5) layers result in asymmetric column intensity, the contrast difference between neighbour columns is much less than that in a single layer and our simulation demonstrates such subtle difference shown in three layers was not corresponding to the real STEM image. In addition, atomically resolved EELS mapping was performed to identify the elements unambiguously (see Supplementary Fig. S2 ). Using the reference spectra of the Mo N 2,3 edge and W O 2,3 edge, 2D EELS chemical maps for each element were obtained. They indeed confirmed the manifestation of W and Mo atoms, respectively, as the brighter and less bright spots in the ADF image. Figure 2: Discrimination of Mo and W atoms. ( a ) An ADF image of a Mo 1− x W x S 2 single layer with x =0.2 (filtered), in which the atomic positions of sulphur are also visible. ( b , c ) Modelled structure and simulated ADF image (red: Mo, blue: W, yellow: S). Note that the two sulphur atoms are overlapped with a small inclination of (5° in x axis and 6° in y axis). ( d , e ) Profiles of the experimental and simulated ADF counts for lines indicated in a and c . They confirm the W, Mo and 2S atomic sites, that is, the brighter spots correspond to W and the less bright ones to Mo. Note that a fast Fourier transform smoothing applied might result in an image contrast variation at most 4%. An absorption potential approach using a multislice calculation with the Mactempas software is used in the simulation profile. Scale bar, 0.5 nm. Full size image Next, we attempted to investigate the distributions of W and Mo atoms quantitatively within a single Mo 1− x W x S 2 layer. Generally, the alloys (or compounds) imply two or more elements mixed in a solid solution. Whether the structure is ordered or disordered depends on the atomic configuration, and in particular, the neighbouring species. In the present case, the sulphur atoms are located at the original trigonal lattice, and the Mo and W atoms share the metal sites (see Fig. 2b ). The ratio of the coordination number of Mo around W and that of W around Mo should be quantified to give the total coordination number. Note that we ignore the S sites in this study. We take the total coordination number as six, because only the in-plane structure is considered. The atomic sites of the stacked adjacent layers are disregarded. Quantitative alloying degree determination of Mo and W atoms The quantitative analysis of the atomic distributions is presented in Fig. 3 . The number of heteroatoms in neighbouring sites can be counted for all the atoms except for them at rims of the image (shown as a rectangle). 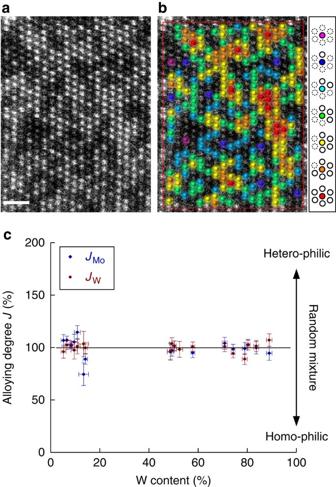Figure 3: Quantitative analysis of atomic distributions. (a) Example for ADF image of Mo1−xWxS2single layer (x=0.5). The W atoms are shown in different colours on the same image (b): purple, blue, light blue, green, yellow, orange and red for six-, five-, four-, three-, two-, one- and zero-coordinate sites. (c) The alloying degreesJWandJMothus observed throughout the wide range of W contents are close to 100%, which indicates a random mixture. Taking into consideration the statistical distribution of W and Mo atoms in a layer, the error bars for the content and alloying degree were calculated. The error bar results for content and alloying degree depend directly on a sample size showing bigger error values for samples with smaller size. Scale bar, 1 nm. Figure 3a shows an example of a Mo 1– x W x S 2 layer ( x =0.5). As seen in the example of Fig. 3b , W atoms with six neighbouring Mo atoms are coloured purple. Similarly, blue, light blue, green, yellow, orange and red signify W atoms with five, four, three, two, one and zero Mo coordination, respectively. The total sum of these coloured atoms gives the value of the alloying degree ‘ J ’ for W atoms as [32] Figure 3: Quantitative analysis of atomic distributions. ( a ) Example for ADF image of Mo 1− x W x S 2 single layer ( x =0.5). The W atoms are shown in different colours on the same image ( b ): purple, blue, light blue, green, yellow, orange and red for six-, five-, four-, three-, two-, one- and zero-coordinate sites. ( c ) The alloying degrees J W and J Mo thus observed throughout the wide range of W contents are close to 100%, which indicates a random mixture. Taking into consideration the statistical distribution of W and Mo atoms in a layer, the error bars for the content and alloying degree were calculated. The error bar results for content and alloying degree depend directly on a sample size showing bigger error values for samples with smaller size. Scale bar, 1 nm. Full size image where P observed is defined as the ratio of the averaged Mo coordination number to the total coordination number (six), and P random is the atomic ratio of Mo in the examined layer (see also the Supplementary Methods section). If there is no preference for Mo or W atoms at the neighbouring sites of W atoms, J W should be 100%. J W <100% means a homophilic configuration, while J W >100% implies a heteroatom-rich configuration. J Mo can also be estimated from the same ADF image. For the particular case shown in Fig. 3a , J Mo =95% and J W =100%, with a W content of 58%. More than 3,000 atoms were thus counted for the wide range of specimen contents ( x =0.2–0.8), and the results are summarized in Fig. 3c . It is clear that J W and J Mo are very close to 100% for all the W contents, although the values are rather scattered for lower W contents. This figure indeed proves the random alloying of Mo 1– x W x S 2 layers. No indication of phase separation or segregation can be found. The results overlooking the 2D structures shown in Supplementary Fig. S3 with different compositions indeed indicate the random alloying without any ordering structure. A theoretical study has also predicted the substitutional doping in a certain range of mixed dichalcogenide [33] . It is in fact worthy to stress here that the two extreme methods ensure a similar structure and support each other. Although alloying is a general phenomenon, there is still a lack of experimental approaches for studying the atomic distributions quantitatively. The alloying behaviour of the surfaces of three dimensional (3D) materials can be also investigated by scanning tunnelling microscopy (STM) [34] , [35] . Discrimination of S and Se atoms on the surface of a 2D solid solution WSeS with STM has also been reported [36] . STM is thus an alternative method to investigate mostly the chalcogenide top layer. Especially in low-dimensional materials, the heteroatomic distribution is a key issue, as this largely governs their properties. For example, the catalytic behaviour of bimetallic nanoparticles is indeed dependent on the atomic distributions of noble metals such as Pt and Au. The present study provides a direct method for visualizing the atomic distributions in such nanostructured materials. The single-layer material presented here is an ideal case. In the case of 3D structures, this method would not be completely suitable for studying the relationships between stacked layers, as this would require 3D information on the atomic coordinates. Even though our dichalcogenide specimens are most intriguing in the single-layered structure because of the possible applications for devices with a direct bandgap, the characterization method may be extended to 3D structures if a similar technique for 3D microscopy [37] can be applied in future. Specimen growth Single crystals of Mo 1− x W x S 2 solid solutions were grown by the chemical-vapour transport method using the starting materials Mo (purity 99.99%), W (purity 99.95%) and S (purity 99.999%). Before the crystal growth, the powdered compounds were prepared from the elements by reaction at 1,000 °C for 10 days in an evacuated quartz ampoule. The mixture was heated slowly to avoid any explosions due to the strongly exothermic reaction between the elements. For single-crystal growth, the mixture materials and Br 2 (≈8 mg cm −3 ) were placed in a quartz ampoule, which was chilled in liquid nitrogen, evacuated to ≈5 × 10 −6 mbar and sealed. On the first day, the growth ends of the ampoules were set at a higher temperature than the charge zone to remove nucleating centres from the growth zone. The furnace was then equilibrated to give a constant temperature across the reaction tube and was programmed over 24 h to produce the temperature gradient at which single-crystal growth would take place. Optimum crystal growth was achieved with the charge zone maintained at 1,030 °C and the growth zone at 980 °C. After 20 days, the furnace was allowed to cool down slowly (40 °C h −1 ). The ampoule was opened when it reached room temperature, and the crystals were removed and rinsed in alcohol. The crystals had the shape of thin-layer plates with thicknesses and surface areas ranging from 20 to 1,000 μm and 20 to 100 mm 2 , respectively. STEM-ADF, EDX and EELS experiments Two STEMs were used for ADF imaging. A JEM-ARM200F with a CEOS corrector was operated at 80 kV and a JEM-2100F with a DELTA corrector at 60 kV. The scanning rate is typically 38 μs per pixel and an image consists of 512 × 512 pixels. A Gatan GIF Quantum equipped with the JEM-2100F was used for EELS analysis. The probe size is 0.1 nm with 20-pA probe current. The energy resolution of the instrument is ~0.35 eV at the full-width half-maximum of elastic peak. The typical EELS acquisition time was 0.01–0.05 s for each spectrum. The ADF image ( Fig. 2 ) was recorded at a convergence angle of α =30 mrad and an inner angle of β 1 =45–55 mrad. The EDX was equipped with the JEM-ARM200F. The collection efficiency for EDX signals is smaller than 0.1 sr. How to cite this article : Dumcenco, D.O. et al . Visualization and quantification of transition metal atomic mixing in Mo 1− x W x S 2 single layers. Nat. Commun . 4:1351 doi: 10.1038/ncomms2351 (2013).